Microwave synthesizer using an on-chip Brillouin oscillator Low-phase-noise microwave oscillators are important to a wide range of subjects, including communications, radar and metrology. Photonic-based microwave-wave sources now provide record, close-to-carrier phase-noise performance, and compact sources using microcavities are available commercially. Photonics-based solutions address a challenging scaling problem in electronics, increasing attenuation with frequency. A second scaling challenge, however, is to maintain low phase noise in reduced form factor and even integrated systems. On this second front, there has been remarkable progress in the area of microcavity devices with large storage time (high optical quality factor). Here we report generation of highly coherent microwaves using a chip-based device that derives stability from high optical quality factor. The device has a record low electronic white-phase-noise floor for a microcavity-based oscillator and is used as the optical, voltage-controlled oscillator in the first demonstration of a photonic-based, microwave frequency synthesizer. The synthesizer performance is comparable to mid-range commercial devices. The generation of low-phase-noise radio, microwave and optical signals relies upon resonant devices that feature large storage times or equivalently high-Q factors [1] , [2] . Maintaining large storage time, in compact or integrated circuits, becomes increasingly challenging with decreasing size and increasing frequency [3] , [4] . These two scaling laws of performance create challenges for compact or integrated microwave and millimeter-wave sources, wherein performance (in terms of phase noise at a given offset frequency) steadily degrades with increasing oscillation frequency [4] . As a result, state-of-the-art microwave oscillators are larger, discrete devices based on dielectric resonators [5] . The introduction of optical fibre for long-distance communication had a positive impact on the frequency scaling side of this problem. First, the distribution of microwaves over optical fibre has led to remarkable progress on transfer of low-phase-noise microwaves onto optical carrier waves [3] , [6] . Second, fibre delay lines provided a way to create long storage time with no frequency-dependent attenuation in hybrid optoelectronic oscillators [7] . These high-performance optoelectronic oscillators represented a paradigm shift in the generation of microwaves and were followed by optical resonator-based versions that employed an optical microcavity to achieve the requisite oscillator storage time [8] , [9] . Generally, the ability to achieve long storage times in compact, high-Q resonators has experienced a major leap forward during this same period [10] , [11] , [12] , [13] , [14] , [15] . On another front, both fibre and optical resonators have also been applied to create microwaves by heterodyne of coherent laser lines [16] , [17] . In this case, co-oscillation occurs within the same cavity so that a high level of common-mode noise suppression leads to good performance microwave generation [16] , [18] . Sideband injection locking in a master-slave laser configuration has also been applied to enable broadband multiplication of a supplied electronic microwave signal [19] . A remarkable, recent advance has been the introduction of optical dividers in the form of frequency combs to create record low close-to-carrier phase-noise microwave signal sources [20] . Frequency combs have previously been applied to stabilize optical carrier frequencies for distribution of microwaves over optical fibre [21] , [22] , [23] , however, in this new approach an optical signal serves as the root for the ultra-high-stability microwave signal itself. Although the technique is complex, emerging technologies like frequency microcombs [24] , [25] and compact reference cavities [26] , [27] , [28] , [29] could one day lead to chip-based photonic microwave sources that exceed the performance of the best electronic sources. In a related development, microcavity-based microcombs and parametric oscillators are providing a new way to synthesize microwaves directly [30] , [31] , [32] , [33] , [34] , [35] . Although the performance is well off from the optical divider approach, the method is less complex. In this work, we report the application of cascaded Brillouin oscillation to microwave frequency synthesis at a level comparable to mid-range commercial, all-electrical synthesizers. Although fibre-based Brillouin lasers have been studied for microwave generation [36] , [37] , [38] , [39] , [40] , the present device is the first chip-based Brillouin microwave source. Moreover, the device has a record low-white-phase-noise floor (−160 dBc Hz −1 ) for any microcavity-based microwave source (even including non-Brillouin-based methods). It can also generate coherent microwave power in excess of 1 mW without any optical or radio frequency (RF) amplification, a significant simplification as it eliminates the need for microwave amplification stages after the photodetector. Moreover, being chip-based devices, the current sources offer integration opportunities for control and additional functions. Microwave generation using chip-based Brillouin lasers An ultra-high-Q planar silica-on-silicon disk resonator [15] is used for cascaded Brillouin oscillation and microwave generation. Microcavity-based Brillouin lasers have only recently been demonstrated [41] , [42] , [43] . The present devices are silicon-chip based and they feature very high coherence and high quantum efficiency [15] , [44] . Both high-power and low-phase-noise microwave generation from the disk resonator are achieved by cascaded stimulated Brillouin lasing and subsequent photomixing of pairs of Brillouin laser as illustrated in Fig. 1a . A narrow-linewidth fibre laser (effective linewidth 1 kHz) is used as the pump laser and is coupled to the disk resonator (see photomicrograph in Fig. 1b ) through a taper fibre technique [45] . The size of the disk resonator (~6 mm) is carefully designed such that the free spectral range of the cavity matches the Brillouin gain shift [15] , [44] . Once the coupled pump power reaches the stimulated Brillouin threshold, the first-order Stokes wave is excited in the backward direction and is routed through a fibre circulator to an optical spectral analyser, a monitor photodetector (bandwidth 125 MHz) and a fast photodetector (bandwidth 50 GHz). Further increase of the pump power leads to cascaded Brillouin lasing, for example, 9th-order Stokes has been demonstrated in our previous work [44] . These cascaded lines feature Schawlow–Townes noise <0.1 Hz 2 Hz −1 (refs 15 , 44 ) and low technical frequency noise. As a result, they are suitable for high-stability microwave synthesis by photomixing. Fine control of this frequency is possible by adjustment of the pump frequency using acousto-optic modulation. The detected Brillouin laser can therefore function as the voltage-controlled oscillator (VCO) in a microwave synthesizer as illustrated in Fig. 1c . 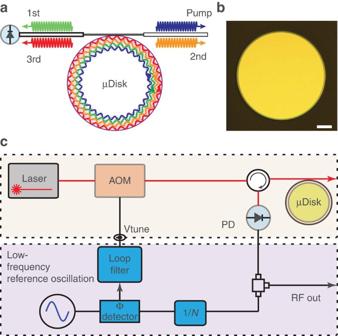Figure 1: Explanation of microwave synthesizer using chip-based Brillouin laser. (a) A Brillouin microwave oscillator showing pump (blue) and second Stokes (orange) waves, and the first (green) and third (red) Stokes waves incident on the detector for microwave generation. (b) Photograph of an ~6 mm ultra-high-Q planar silica disk resonator on a silicon chip. Scale bar, 1 mm. (c) Block diagram for a closed-loop Brillouin microwave oscillator. The open-loop Brillouin microwave oscillator (shown in the upper dashed box) functions as a voltage-controlled photonic oscillator. All hardware in the upper dashed box replaces an electrical VCO in a conventional electrical synthesizer. Components in the upper box include a pump laser, acousto-optic modulator (AOM), circulator, high-speed detector and ultra-high-Q disk resonator. PD, photodetector. Figure 1: Explanation of microwave synthesizer using chip-based Brillouin laser. ( a ) A Brillouin microwave oscillator showing pump (blue) and second Stokes (orange) waves, and the first (green) and third (red) Stokes waves incident on the detector for microwave generation. ( b ) Photograph of an ~6 mm ultra-high-Q planar silica disk resonator on a silicon chip. Scale bar, 1 mm. ( c ) Block diagram for a closed-loop Brillouin microwave oscillator. The open-loop Brillouin microwave oscillator (shown in the upper dashed box) functions as a voltage-controlled photonic oscillator. All hardware in the upper dashed box replaces an electrical VCO in a conventional electrical synthesizer. Components in the upper box include a pump laser, acousto-optic modulator (AOM), circulator, high-speed detector and ultra-high-Q disk resonator. PD, photodetector. Full size image The Brillouin shift in the silica disk cavity is around 10.8 GHz (ref. 44 ), so that microwave generation from around 10.8 to 86 GHz is feasible in the present device by photomixing pairs of the cascaded Brillouin lines. We have focused on the generation of K-band (~21.5–21.8 GHz) microwave signals by photomixing the first and third Stokes lines. Operationally, these lines feature high coherence with very low Schawlow–Townes noise and technical noise; they also provide high-power levels and propagate in the same direction. It is important to note that besides the common-mode noise suppression that occurs upon photomixing because the Brillouin laser lines share a common laser cavity, combinations of laser lines that share the same optical path (that is, odd–odd and even–even Stokes pairs) also enable cancellation of any optical-path length jitter effects. Phase noise of optical VCO To measure the phase noise of the K-band microwave signal, a phase-noise analyser (Rohde-Schwartz FSUP Signal Source Analyzer) is used. 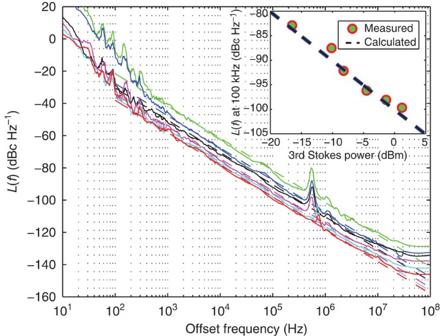Figure 2: Power dependence of microwave phase noise. The microwave signal is produced by photomixing the first and third Stokes lines on a high-speed detector. The output optical power of the third Stokes line is increasing from top to bottom curves (−16.5, −10.2, −8.2, −4.5, −1.4 and 1.2 dBm, respectively). The phase noise shows 1/f2dependences for five decades from 200 Hz to 20 MHz. The dashed lines are 1/f2fits to the measured phase-noise spectra. Inset: plot showing inverse power dependence of the phase noise of the Brillouin microwave signal (100 kHz offset frequency) on the optical power of the third Stokes line. Circles, measured values; dashed line, calculated values based upon the Schawlow–Townes formula. Figure 2 shows the single-sideband phase noise ( L ( f )) of a 21.7-GHz signal generated using the first and third Stokes laser lines for a series of output optical power levels of the 3rd Stokes (−16.5, −10.2, −8.2, −4.5, −1.4 and 1.2 dBm from upper to lower curves). Significantly, the phase noise of this signal has 1/ f 2 dependence over five decades (200 Hz to 20 MHz), which corresponds to white frequency noise. Moreover, this 1/ f 2 noise has an inverse dependence on the third Stokes laser line power as shown in the inset to Fig. 2 (phase noise is measured at 100 kHz frequency offset, and power is varied by changing the pump power). The inset of Fig. 2 also shows a calculated phase noise based on the Schawlow–Townes frequency noise of the third Stokes line power. For a Brillouin laser, the two-sided Schawlow–Townes frequency noise [44] can be rewritten as: Figure 2: Power dependence of microwave phase noise. The microwave signal is produced by photomixing the first and third Stokes lines on a high-speed detector. The output optical power of the third Stokes line is increasing from top to bottom curves (−16.5, −10.2, −8.2, −4.5, −1.4 and 1.2 dBm, respectively). The phase noise shows 1/ f 2 dependences for five decades from 200 Hz to 20 MHz. The dashed lines are 1/ f 2 fits to the measured phase-noise spectra. Inset: plot showing inverse power dependence of the phase noise of the Brillouin microwave signal (100 kHz offset frequency) on the optical power of the third Stokes line. Circles, measured values; dashed line, calculated values based upon the Schawlow–Townes formula. Full size image where P is output power of the Brillouin laser, τ ( τ ex ) is the total (external) cavity photon life time, c is the speed of light, n is the refractive index of silica and V a is the sound velocity in silica. This equation gives the limit of the Schawlow–Townes noise formula [44] when the number of thermal quanta of the Brillouin phonons is far greater than unity, which is the case for measurements taken at room temperature (thermal quanta=569). It is important to note that the Schawlow–Townes noise is independent of both the pump frequency and the Brillouin frequency. As a result, at an equivalent power level, the phase-noise levels measured in Fig. 2 would be expected if the pump frequency was higher resulting in a higher-frequency Brillouin shift. For the calculation of the Shawlow–Townes noise, measured cavity τ of τ =28 ns and τ ex =34 ns are used (that is, no free parameters are used), and L ( f )=10log . Here is the one-sided power spectral density of phase noise and is related to the two-sided power spectral density of frequency noise as: . Because the output optical power of the first Stokes line varies over 2.5–5.0 dBm from the upper to lower measurement curves (that is, power levels much greater than for the third Stokes wave), the Schawlow–Townes noise of the first Stokes line is not expected to be a significant component of noise in the photomix-generated carrier wave. Indeed, the good agreement between the measurement values and calculation in the inset of Fig. 2 shows that the phase noise of the Brillouin microwave signal is mainly contributed by the Schawlow–Townes noise of the third Stokes line. As a general comment relevant to the discussion of phase noise in the introduction, the results in Fig. 2 confirm that the very high-Q factor of the Brillouin laser (high storage time) leads to the low-microwave phase noise upon photomixing of the Stokes laser lines. Ultimately, the cascade process sets the limit of phase noise in these devices (see Supplementary Note 1 ). Finally, at low-offset frequencies in Fig. 2 , the phase noise exhibits a non-Schawlow–Townes component. Although Brillouin lasers suppress technical phase noise from the pump [44] , [41] , it is possible that this noise is contributed by the pump. It is also possible that this noise is environmental related. The closed-loop control described in the next section suppresses this noise. Phase-locked operation of oscillator The Brillouin microwave oscillator can be operated in two distinct ways: open loop (no feedback control) and closed loop (phase-lock-loop control). In open-loop operation, the first and third Stokes lines from the resonator are directly photomixed on a fast photodetector with no other control. This is the method used for the spectra in Fig. 2 . Alternatively, the centre frequency of the free-running Brillouin microwave oscillator can be finely varied in the range of 100 s kHz to a few MHz, by adjusting the pump laser frequency either through a piezo control of the pump laser cavity or with an external acousto-optic modulator. Thus, the Brillouin oscillator constitutes a VCO, and the device can be configured into a phase-lock-loop control design (that is, closed-loop operation). Phase-lock-loop control of optically generated microwave tones has been previously accomplished by reference to a high-performance microwave reference [46] , [47] , [48] . In these earlier works, the objective was to use the the high-stability microwave electrical reference to stabilize the optical generated tone. In the present case, the original microwave tone from the open-loop stimulated Brillouin scattering (SBS) oscillator is already of sufficient stability at shorter times (higher offset frequencies), so that the phase-lock-loop (PLL) is used only to obtain long-term stability. Moreover, the loop control does not use another microwave oscillator to achieve stability, but rather a low-frequency quartz oscillator via electrical frequency division. Indeed, the divider used here not only allows stabilization using a low-frequency reference oscillator but also converts the SBS microwave signal into nearly any microwave signal frequency <21.8 GHz. As a result, this device constitutes a microwave synthesizer with performance comparable to good commercial electrical synthesizers. The essential elements of the SBS microwave synthesizer are shown in the experimental schematic of Fig. 3a . The synthesizer is analysed by a phase-noise analyser and an Allan deviation tester (ADEV), and a mutual time base is shared between the frequency reference, phase-noise analyser and the ADEV. 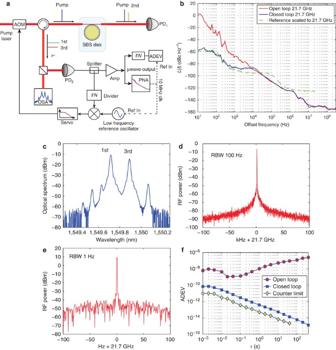Figure 3: Performance of the synthesizer for both open and closed-loop operation. (a) Experimental schematic for the closed-loop Brillouin microwave oscillator. AOM, acouto-optic modulator;f/N, frequency divider; PD, photodetector; OSA, optical spectrum analyzer. A mutual time base is shared between the phase-noise analyser (PNA), low-frequency reference oscillator and the ADEV. (b) Open-loop (red curve) and closed-loop (blue curve) single-sideband phase noise of the Brillouin oscillator at 21.7 GHz. The green dashed line is the phase noise of the reference oscillator scaled up to 21.7 GHz. (c) Optical spectrum of the 1st-Stokes and 3rd-Stokes laser emission lines. The pump wave is also visible, but is weak on account of propagation opposite to the direction of the 1st and 3rd Stokes lines. Also visible is the 5th Stokes line in the spectrum as well as the first anti-Stokes wave. (d) RF spectrum of an open-loop Brillouin oscillator at 21.7 GHz. The span is 200 kHz and the resolution bandwidth (RBW) is 100 Hz. (e) RF spectrum of a closed-loop Brillouin oscillator at 21.7 GHz. The span is reduced to 200 Hz and the RBW is 1 Hz. (f) Allan deviation (ADEV) of the Brillouin microwave oscillator. Circle markers represent the open-loop operation, square markers represent the residual Allan deviation for the close-loop operation and the diamond markers give the counter limit. Figure 3: Performance of the synthesizer for both open and closed-loop operation. ( a ) Experimental schematic for the closed-loop Brillouin microwave oscillator. AOM, acouto-optic modulator; f / N , frequency divider; PD, photodetector; OSA, optical spectrum analyzer. A mutual time base is shared between the phase-noise analyser (PNA), low-frequency reference oscillator and the ADEV. ( b ) Open-loop (red curve) and closed-loop (blue curve) single-sideband phase noise of the Brillouin oscillator at 21.7 GHz. The green dashed line is the phase noise of the reference oscillator scaled up to 21.7 GHz. ( c ) Optical spectrum of the 1st-Stokes and 3rd-Stokes laser emission lines. The pump wave is also visible, but is weak on account of propagation opposite to the direction of the 1st and 3rd Stokes lines. Also visible is the 5th Stokes line in the spectrum as well as the first anti-Stokes wave. ( d ) RF spectrum of an open-loop Brillouin oscillator at 21.7 GHz. The span is 200 kHz and the resolution bandwidth (RBW) is 100 Hz. ( e ) RF spectrum of a closed-loop Brillouin oscillator at 21.7 GHz. The span is reduced to 200 Hz and the RBW is 1 Hz. ( f ) Allan deviation (ADEV) of the Brillouin microwave oscillator. Circle markers represent the open-loop operation, square markers represent the residual Allan deviation for the close-loop operation and the diamond markers give the counter limit. Full size image The optical spectrum of the generated Stokes lines in the back-propagating direction is shown in Fig. 3c and includes the first and third Stokes lines that are used to generate the microwave tone of the present work. The incident optical power levels of the first and third Stokes lines on the high-speed photodiode are 3.7 and 1.7 mW, respectively (the coupled optical pump power to the microresonator was 31 mW). For comparison purposes, the open- and closed-loop phase-noise spectra are presented in Fig. 3b together with the scaled-up phase noise of the low-frequency reference oscillator. Phase-noise levels (open loop) of −90 dBc Hz −1 at 10 kHz offset and −110 dBc Hz −1 at 100 kHz are obtained for the 21.7 GHz carrier. The measured white-phase-noise floor of the oscillator (−156 dBc Hz −1 >100 MHz) is a record for a microcavity-based microwave source by several orders of magnitude [9] , [30] , [35] . The calculated shot noise floor is −158 dBc Hz −1 for the 21.7 GHz carrier, with 2.2 mA average photocurrent and a generated RF power of −15.5 dBm, and is in good agreement with the measured result. Using another device, both a higher RF power of 2.9 dBm (1.9 mW, no optical or RF amplification) and yet lower white-phase-noise floor of −160 dBc/Hz were obtained. These results are within 19 dB of the very lowest white-phase-noise floors recently demonstrated using high-performance frequency combs and high-power photodiodes [49] . Further details on this measurement as well as the power calculations themselves are provided in the Supplementary Note 2 . For closed-loop operation, an integer frequency divider (1/32) is used to divide the free-running microwave carrier to 678 MHz for phase comparision with a low-frequency reference oscillator at 678 MHz. The blue curve in Fig. 3b shows the phase noise of the closed-loop Brillouin oscillator. The close-to-carrier phase noise is now greatly reduced. The phase noise of the frequency reference is also shown in Fig. 3b as the green dashed line. A factor of 20 × log32=30 dB has been added to this line to account for phase-noise scaling with frequency, and thereby enable comparison with the phase noise of the closed-loop oscillator. As expected, for low-offset frequencies, the closed-loop oscillator tracks the scaled-up reference noise. The corresponding RF spectra for the open-loop (span 200 kHz and resolution bandwidth 100 Hz) and closed-loop (span 200 Hz and resolution bandwidth 1 Hz) oscillators are given in Fig. 3d , respectively. To characterize the long-term frequency stability of the Brillouin oscillator, ADEV measurements were carried out for open-loop and closed-loop operation using gate times from 1 to 400 s. The measurement results (normalized to the Brillouin oscillator frequency) are shown in Fig. 3f . For these measurements, a sub-harmonic (1/256) at 84.6 MHz of the Brillouin oscillator is measured, as the maximum input frequency of the ADEV is 400 MHz. It can be seen that the long-term drift of the open-loop VCO is greatly suppressed. More than 80 dB reduction of the ADEV (with respect to the 10-MHz mutual time base) is obtained at 400 s gate time. Also, a residual Allan Deviation of 5 × 10 −13 is achieved at 1 s. Overall, the closed-loop Brillouin oscillator has low phase noise at both close-to-carrier and high-offset frequencies. In fact, the phase-noise level demonstrated here is between a mid-range (Agilent N5183A MXG, phase noise of −97 dBc/Hz at 100 kHz offset for 20 GHz carrier; Data Sheet, Literature number 5989-7572EN) and high-performance (Agilent E8257D PSG, phase noise of −111 dBc/Hz at 100 kHz offset for 20 GHz carrier; Data Sheet, Literature number 5989-0698EN) commercial electrical microwave synthesizers. Frequency synthesizer operation RF frequency synthesis derived from the low-noise closed-loop Brillouin oscillator was also demonstrated. This is done by using a (fractional or integer) frequency divider to divide the closed-loop Brillouin oscillator at 21.7 GHz to different frequencies. A series of the phase-noise spectra using different division ratios ( f / N ; N =32, 256, 512, 1,024 and 2,048) is shown in Fig. 4a . Generally, the single-sideband phase noise L ( f ) will drop 20log N dB upon frequency division. Thus, RF frequency synthesis at arbitrary frequencies up to 22 GHz is possible based on the low-noise K-band Brillouin oscillator. The time-domain traces are shown in Fig. 4b for 2.7 GHz, 1.35 GHz and 678 MHz, measured using an oscilloscope with 4 GHz bandwidth. 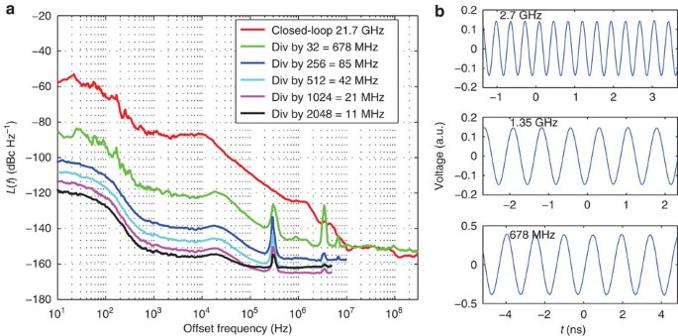Figure 4: RF frequency synthesis by the K-band low-noise Brillouin microwave oscillator. (a) Phase noise of a series of RF frequencies generated by frequency division (Div) in the synthesizer. (b) Typical sine-wave, time-domain traces of the synthesizer output at 2.7 GHz, 1.35 GHz and 678 MHz (from top to bottom). All frequencies lower than the base oscillator frequency of 21.7 GHz are possible, and the traces selected here were limited by the bandwidth of oscilloscope (4 GHz). Figure 4: RF frequency synthesis by the K-band low-noise Brillouin microwave oscillator. ( a ) Phase noise of a series of RF frequencies generated by frequency division (Div) in the synthesizer. ( b ) Typical sine-wave, time-domain traces of the synthesizer output at 2.7 GHz, 1.35 GHz and 678 MHz (from top to bottom). All frequencies lower than the base oscillator frequency of 21.7 GHz are possible, and the traces selected here were limited by the bandwidth of oscilloscope (4 GHz). Full size image Out-of-loop Allan deviation Finally, closed-loop operation of the Brillouin oscillator was also possible by referencing to a fixed-frequency, ultra-low-noise oven-controlled crystal oscillator (OCXO) at 400 MHz. 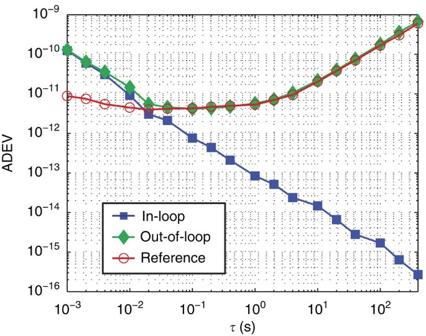Figure 5: Allan deviation measurements. The Brillouin microwave oscillator (21.7 GHz) is phase locked to an ultra-low-noise OCXO at 400 MHz as reference. The blue square markers are the residual Allan deviation (ADEV) of the Brillouin microwave oscillator with regard to the reference OCXO. The green diamond markers are the out-of-loop Allan deviation, measured against a second low-noise OCXO at 10 MHz. The red circle markers are the Allan deviation of the reference OCXO at 400 MHz measured against the second OCXO at 10 MHz. Figure 5 shows the Allan deviation measurements normalized to the Brillouin oscillator frequency. The blue square markers are the residual ADEV of the Brillouin microwave oscillator with regard to the reference OCXO. For a more rigorous measurement, we also measure the out-of-loop Allan deviation of the closed-loop VCO using a second independent ultra-low-noise OCXO (10 MHz). The green diamond markers are the out-of-loop ADEV and the red circle markers are the ADEV of the reference OCXO at 400 MHz measured against the second OCXO at 10 MHz. The out-of-loop ADEV tracks the 400 MHz reference for τ >0.03 s. Thus, the out-of-loop ADEV is reference-limited, and an out-of-loop ADEV level of 5 × 10 −12 at 1 s gate time is demonstrated. Figure 5: Allan deviation measurements. The Brillouin microwave oscillator (21.7 GHz) is phase locked to an ultra-low-noise OCXO at 400 MHz as reference. The blue square markers are the residual Allan deviation (ADEV) of the Brillouin microwave oscillator with regard to the reference OCXO. The green diamond markers are the out-of-loop Allan deviation, measured against a second low-noise OCXO at 10 MHz. The red circle markers are the Allan deviation of the reference OCXO at 400 MHz measured against the second OCXO at 10 MHz. Full size image In this work, we have demonstrated a microwave synthesizer with commercial-level frequency stability using a compact, on-chip Brillouin laser VCO. The combined demonstrations show that the Brillouin VCO can operate as a direct replacement for conventional electronic VCO devices. Significantly, the phase noise of the Brillouin VCO does not degrade with increasing frequency as compared with electronic devices. This is because the phase noise contributed by the underlying Stokes lines (assuming constant power in each line) is not sensitive to order or to pump frequency. Also, by operating the Brillouin at shorter pump wavelengths or by operating on higher-order Stokes lines, the base frequency of the synthesizer can be readily boosted. For example, by operation with a green pump (doubled yttrium aluminum garnet laser), the base frequency would be boosted to beyond 60 GHz using the same Stokes 1 to Stokes 3 photomixing configuration demonstrated here (again with no degradation in phase-noise performance). Also, by operation on the 1–5 or 1–7 Stokes combinations, millimeter-wave generation well beyond 100 GHz is feasible. Likewise, electronic dividers have been demonstrated to these frequencies [50] , thereby making the possibility of high-performance millimeter-wave synthesizers possible using this approach. It is important to note that such millimeter-wave synthesizers would be predicted to produce X-band signals with significantly lower phase noise than what has even been demonstrated here. This is because the divider process quadratically improves the phase noise. For example, by only maintaining the Schawlow–Townes noise at shorter pump wavelengths, the predicted X-band (~10 GHz) phase-noise level would be −130 dBc Hz −1 at 100 kHz offset upon division of a 90-GHz SBS-generated base frequency. Ultimately, the current limit to phase noise in these devices is the onset of cascade to higher-order Stokes lines. If this process could be forestalled through, for example, judicious cavity dispersion control, then much lower phase-noise levels than what has been demonstrated here are possible. How to cite this article: Li, J. et al . Microwave synthesizer using an on-chip Brillouin oscillator. Nat. Commun. 4:2097 doi: 10.1038/ncomms3097 (2013).